Carbon precipitation from heavy hydrocarbon fluid in deep planetary interiors The phase diagram of the carbon–hydrogen system is of great importance to planetary sciences, as hydrocarbons comprise a significant part of icy giant planets and are involved in reduced carbon-oxygen-hydrogen fluid in the deep Earth. Here we use resistively- and laser-heated diamond anvil cells to measure methane melting and chemical reactivity up to 80 GPa and 2,000 K. We show that methane melts congruently below 40 GPa. Hydrogen and elementary carbon appear at temperatures of >1,200 K, whereas heavier alkanes and unsaturated hydrocarbons (>24 GPa) form in melts of >1,500 K. The phase composition of carbon-hydrogen fluid evolves towards heavy hydrocarbons at pressures and temperatures representative of Earth’s lower mantle. We argue that reduced mantle fluids precipitate diamond upon re-equilibration to lighter species in the upwelling mantle. Likewise, our findings suggest that geophysical models of Uranus and Neptune require reassessment because chemical reactivity of planetary ices is underestimated. Methane is one of the most abundant hydrocarbon molecules in the universe, and along with water and ammonia comprises a significant part of the icy giant planets (Uranus and Neptune) and their satellites [1] , [2] . The chemical composition of planetary ices and possible chemical reactions within deep interiors of these planets are critical for understanding their thermal, magnetic and electrical properties [3] , and represent necessary input information for theoretical modelling [4] . Also, the behaviour of hydrocarbons as a part of reduced carbon-oxygen-hydrogen fluid within the deep Earth is of particular interest as oxygen fugacity below the wustite–magnetite buffer is likely to shift fluid phase composition from CO 2 –H 2 O to CH 4 –H 2 O in the simplest modelling [5] , [6] , [7] , [8] . However, phase relations in the C–H system are poorly understood even at relatively low pressures. For example, the results of methane melting curve measurements are contradictory and report only up to 4.8 (ref. 9 ) and 6.8 GPa (ref. 10 ). Moreover, theoretical and experimental studies of chemical reactivity of liquid CH 4 differ by several thousand Kelvin [11] , [12] , [13] , [14] . Whether there is a formation of hydrocarbons other than methane, what are the limits of their stability under extreme conditions, and what their role is in deep carbon reservoirs and fluxes of the Earth or icy giant planets remain unanswered questions. Thermodynamic modelling of C–H systems [7] , [15] , as well as ab initio molecular dynamic (MD) computations [12] , [14] , show the rise of stability of heavier hydrocarbons with increasing pressure and temperature. According to MD, methane dissociates to molecular hydrogen and diamond at pressures of >300 GPa and at temperatures of >4,000 K (ref. 12 ). Likewise, such chemical reactions were observed in experiments with laser-heated (LH) diamond anvil cells (DAC), where methane produces carbon, hydrogen and heavier hydrocarbons at temperatures of 2,000–4,000 K and under pressures up to 80 GPa (refs 11 , 13 , 16 , 17 ). On the other hand, shock experiments suggest no chemical reactivity up to 26 GPa and 3,200 K (ref. 18 ). The discrepancy between the results obtained by LH DAC, shockwave, MD and thermodynamics may arise from various assumptions in modelling as well as from kinetic, catalytic and analytical problems in the experiments. Recent advances in resistively heated (RH) and LH techniques allow for better control of P–T conditions in DAC cavity [19] , [20] , as well as for more accurate characterization of the physico-chemical processes than previously possible. Here we report our measurements of the methane melting curve and chemical reactivity of the C–H system up to 80 GPa and 2,000 K using RH and LH DACs. We partly reconcile contradictions between previously reported results, and relate our observations to the processes in planetary interiors. Methane melting Several criteria were employed to recognize melting in the RH DAC experiments. Simultaneous measurements of temperature and pressure revealed discontinuities in P–T paths during the RH, which were followed by abrupt changes in Raman spectra of ν 1 – ν 3 modes ( Supplementary Fig. S1 ). Also, we were able to observe convection motion of small particles (gasket pieces or rubies) imbedded in the sample, as well as a phase boundary marked by different refractive indices of coexisting fluid and solid once the melting temperature was reached. The most accurate measurements of CH 4 melting in LH experiments were found to be through the observations of small vesicles (2–4 μm) of molten material in contact with solid phases. Rounded vesicles reproducibly appear near the rim of an Ir heat absorber foil (coupler) heated with the infrared (IR) laser ( Fig. 1 insert). To verify visual observations of methane liquid state inside the vesicles, several synchrotron-based X-ray diffraction and in situ Raman spectroscopy experiments have been performed (see Methods). Moreover, at temperatures above CH 4 dissociation one can see small graphite particles moving in the vesicle, demonstrating signs of convection. 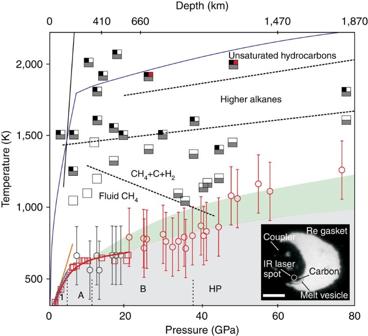Figure 1: C–H system experimental results with CH4as a starting material. Blue triangles represent methane melting after Yagi and Suzuki9and the orange line is after Abramson10. Red squares and circles are our RH and LH melting observations. Red curve is guide to the eye through our RH melting points. Grey circles show LH melting data with coupler temperature at <1,000 K. The error bars for RH melting data are smaller than the symbol size, whereas temperature uncertainties for LH data (±200 K) result mainly from the greybody approximation for sample emissivity (Methods). Grey area shows solid CH4region. Solid phases (1, A, B, HP) and boundaries between them (thin dashed lines) are marked following Chenet al.36Light green area represents CH4melting according to LH experiments. Chemical transformations in C–H fluid are colour-coded by squares (Supplementary Table S2). Blank squares—no chemical reactions, grey—CH4dissociation observed, black—newly formed alkanes, red—C=C bonds detected. Thick dashed lines summarize data for chemical reactivity. Solid black and blue lines are the graphite–diamond equilibrium44and the Earth’s geotherm45, respectively, shown for comparison. The inset is a microphotograph of the LH sample cavity showing the vesicle of molten methane. The scale bar is 25 μm. Figure 1: C–H system experimental results with CH 4 as a starting material. Blue triangles represent methane melting after Yagi and Suzuki [9] and the orange line is after Abramson [10] . Red squares and circles are our RH and LH melting observations. Red curve is guide to the eye through our RH melting points. Grey circles show LH melting data with coupler temperature at <1,000 K. The error bars for RH melting data are smaller than the symbol size, whereas temperature uncertainties for LH data (±200 K) result mainly from the greybody approximation for sample emissivity (Methods). Grey area shows solid CH 4 region. Solid phases (1, A, B, HP) and boundaries between them (thin dashed lines) are marked following Chen et al. [36] Light green area represents CH 4 melting according to LH experiments. Chemical transformations in C–H fluid are colour-coded by squares ( Supplementary Table S2 ). Blank squares—no chemical reactions, grey—CH 4 dissociation observed, black—newly formed alkanes, red—C=C bonds detected. Thick dashed lines summarize data for chemical reactivity. Solid black and blue lines are the graphite–diamond equilibrium [44] and the Earth’s geotherm [45] , respectively, shown for comparison. The inset is a microphotograph of the LH sample cavity showing the vesicle of molten methane. The scale bar is 25 μm. Full size image The results of melting curve measurements are summarized in Fig. 1 and Supplementary Table S1 . RH and LH DAC melting measurements are in agreement if the correction for temperature difference between the coupler temperature (measured using spectroradiometry) and the melt–solid interface temperature is introduced (see Methods). The uncertainties in radiometric temperature measurements are quite large (up to ±200 K), especially at low pressures, where the melting temperatures are lower, which warrants our presentation of the melting line determined in LH experiments as a band rather than a single line. Chemical transformations in C–H fluid Confocal Raman systems (457, 488 nm excitations for LH experiments, and 532 nm for RH) were used to probe the onset of chemical transformations in C–H fluid at high temperatures, as well as to map the samples near the heating spot after quenching, with the assumption that these features could be quenched for ambient temperature studies. This assumption seems reasonable as equilibrium experiments [5] , even with slower quenching rates, are reported to agree with thermodynamic calculations. Our RH experiments show no signs of chemical reactions in solid or liquid methane at pressures up to 24 GPa and temperatures up to 900 K. Methane molecular dissociation was detected at temperatures as low as 1,200–1,500 K. The onset of this reaction is documented by hydrogen formation ( Fig. 2c ). Single, double or triple H–H stretch modes (vibrons) of ~ 4,200–4,700 cm −1 are observed both in quenched samples and at high temperatures ( Supplementary Fig. S2 ). These vibrations are characteristic of CH 4 –H 2 van der Waals compounds [21] , which are formed upon hydrogen escape from the reactor to solid methane surrounding the melt vesicle. 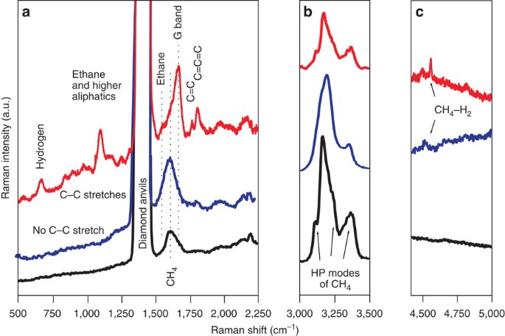Figure 2: Raman spectra of CH4and its reaction products. Synthesis in LH DAC at 48 GPa. Black line shows CH4Raman spectrum before heating. Blue line shows Raman spectrum collected at 1,445 K with evident CH4dissociation. Red line shows Raman spectrum of reaction products collected after heating to 2,000 K. The labels near the curves suggest the assignment of the Raman bands. HP modes of CH4refer to vibrations caused by partial orientational ordering of methane HP phase36. Panelsa–cshow different parts of the spectral range. Figure 2: Raman spectra of CH 4 and its reaction products. Synthesis in LH DAC at 48 GPa. Black line shows CH 4 Raman spectrum before heating. Blue line shows Raman spectrum collected at 1,445 K with evident CH 4 dissociation. Red line shows Raman spectrum of reaction products collected after heating to 2,000 K. The labels near the curves suggest the assignment of the Raman bands. HP modes of CH 4 refer to vibrations caused by partial orientational ordering of methane HP phase [36] . Panels a – c show different parts of the spectral range. Full size image Application of temperatures above 1,500 K results in further CH 4 dissociation and formation of substantial amounts of solid carbon, hydrogen and higher hydrocarbons ( Fig. 2 ; red curve). Increased intensity of H–H stretching is accompanied by the development of molecular H 2 rotational bands at low frequencies with the strongest band near 650 cm −1 (ref. 22 ). The rise in the intensity of the graphite Raman bands correlates with an increase in the proportion of black particles precipitating from the hot convecting fluid as temperature is increased ( Fig. 2a ; red curve). These particles can be observed in situ overgrowing the coupler ( Fig. 1 ; inset). We extracted and documented Raman spectra of these black particles outside DAC ( Fig. 3 ) using a Raman microscope with a very high spatial resolution (see Methods). These spectra provide unambiguous evidence [23] , [24] for carbon precipitation from hydrocarbon fluid. 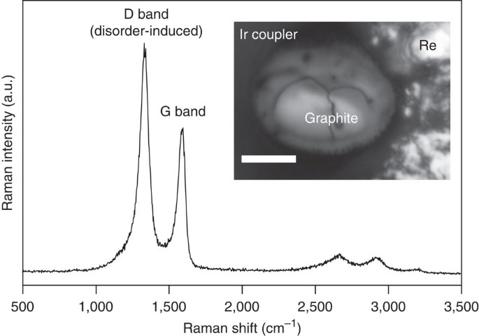Figure 3: Graphite Raman spectrum collected outside the DAC. The spectrum was collected after LH experiment with documented CH4dissociation. D and G bands are in excellent agreement with graphite Raman spectrum23. The inset is a microphotograph of graphite in the LH sample cavity. The sample was recovered after LH to 2,000 K at 7 GPa. The scale bar is 10 μm. Figure 3: Graphite Raman spectrum collected outside the DAC. The spectrum was collected after LH experiment with documented CH 4 dissociation. D and G bands are in excellent agreement with graphite Raman spectrum [23] . The inset is a microphotograph of graphite in the LH sample cavity. The sample was recovered after LH to 2,000 K at 7 GPa. The scale bar is 10 μm. Full size image We investigated the effect of possible hydrogen loss in LH DAC experiments on the observed chemical transformations. Our LH DAC experiments do not suffer from continuous hydrogen depletion as revealed by time-stability experiments ( Supplementary Fig. S2 ). The loss of hydrogen from the hot fluid is mainly temperature-dependent and follows the chemical reactivity. However, we have to admit that C–H systems at high temperature tend to lose hydrogen that is not bound in the C–H fluid; thus, in principle, we cannot rule out that chemical bonding in the C–H system under the studied P–T conditions may be somewhat different if no hydrogen escape had occurred. New Raman peaks ( Fig. 2a ; red curve), which appear at high temperatures at ~ 1,000–1,300 cm −1 and 1,500 cm −1 , correspond to the C–C stretch and C–H bend modes of aliphatic hydrocarbons [25] , respectively. These vibrations are evidences for new hydrocarbons being formed from CH 4 , which is consistent with the previous experimental results by Kolesnikov et al. [16] , who have studied chemical reactivity in the C–H system at pressures of <5 GPa. The sequence of newly formed hydrocarbons starts with ethane and continues further above 1,500 K. Complex changes in C–C stretching and C–H bending spectral regions suggest elongation of the C–C skeleton. LH DAC experiments with nonmetal absorbers (amorphous boron) yielded methane dissociation onset at 2,000 K (P=11 GPa), with subsequent formation of higher alkanes, which is at least 500 K higher than in cases where Ir couplers were used. Indeed, recent ab initio MD calculations also showed that transition metal couplers catalyze chemical transformations in the C–H system as kinetic barriers are decreased if Ir 4 clusters are introduced in the simulation cell [14] . Following high-temperature experiments (~ 2,000 K) at pressures of >24 GPa, Raman spectra of quenched products show very distinct bands in the 1,700–1,800 cm −1 region ( Fig. 2a ; red curve). Based on the system composition, we assign these bands to the formation of unsaturated double-bonded hydrocarbons [25] . As no spectroscopic data are available for carbon-to-carbon double bonds under high pressure, we have collected Raman data of ethylene under pressures up to 16 GPa. Raman frequency shift of presumably double-bonded hydrocarbons upon compression/decompression (1–2 cm −1 GPa −1 ) is in general agreement with our data for ethylene (1.2 cm −1 GPa −1 ). Also, pressure shift of these bands is somewhat lower than that for the C–C stretch mode of single-bonded aliphatic hydrocarbons (~ 3 cm −1 GPa −1 ), which is consistent as the former are stronger. Multiple Raman scans across the quenched samples did not reveal any other chemical reactions. In addition, we have performed LH experiments with C 6 H 14 ( n -hexane) at pressures of 5, 16 and 40 GPa and at temperatures of 1,200–2,000 K. At 5 GPa and 1,200 K, n- hexane decomposed to graphite and methane. In contrast, at 40 GPa and 2,000 K, complex changes occurred in C–C stretching and C–H bending spectral regions, accompanied by the appearance of strong bands in the 1,750–2,250 cm −1 spectral range ( Fig. 4a ). These spectroscopic data strongly suggest formation of complex heavy aliphatic hydrocarbons containing double- and triple-bonded carbons [25] , although their composition and concentration cannot be currently quantitatively determined. Raman spectra of quenched products after LH to 2,000 K at 40 GPa also show very distinct bands in the 4,250–4,500 cm −1 spectral range ( Fig. 4c ), similar to vibrations observed in quenched samples after heating of CH 4 . These bands show that at pressures of 40 GPa, laser heating of n- hexane produced free hydrogen coexisting with heavy hydrocarbons. Therefore, bulk composition of hydrocarbons found after LH are characterized by H/C<2.33 (H/C for n- hexane). 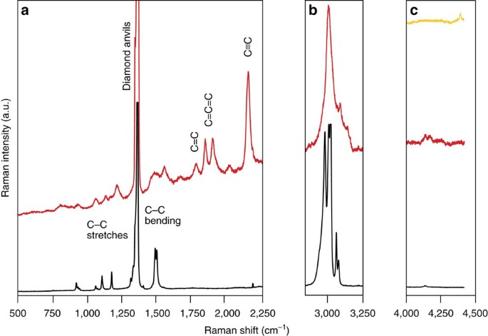Figure 4: Raman spectra ofn-hexane and its reaction products after LH. Red and yellow lines are Raman spectra of quenched reaction products synthesized fromn-hexane at 2,000 K and 40 GPa. Red spectrum was collected at 8 GPa after decompression from 40 GPa (yellow spectrum). Black line isn-hexane Raman spectrum at 8 GPa and 300 K, shown for comparison. Panelsa–cshow different parts of the spectral range. Figure 4: Raman spectra of n- hexane and its reaction products after LH. Red and yellow lines are Raman spectra of quenched reaction products synthesized from n- hexane at 2,000 K and 40 GPa. Red spectrum was collected at 8 GPa after decompression from 40 GPa (yellow spectrum). Black line is n- hexane Raman spectrum at 8 GPa and 300 K, shown for comparison. Panels a – c show different parts of the spectral range. Full size image Figure 1 summarizes experimental data on the CH 4 melting curve and chemical reactivity of the C–H fluid as revealed by Raman spectroscopy of quenched samples synthesized in LH DAC. Methane melts at rather low temperatures compared with other molecular ices such as water [26] , [27] and ammonia [28] . The methane melting curve is significantly lower than the Earth’s average geotherm up to 80 GPa, suggesting that CH 4 is fluid down to at least the middle part of the lower mantle, provided that C–H fluid is present at this depth. Chemical reactions in fluid CH 4 were not observed at low temperatures (<900 K in RH and <1,200 K in LH experiment) and at pressures <40 GPa, suggesting congruent methane melting behaviour. However, one should consider that our Raman technique may not be sufficiently sensitive to detect species at such low concentration levels (<5% mol). This might be the reason for the disagreement between our results and piston-cylinder experimental results [5] as well as thermodynamic prediction [7] , which suggest that a minor admixture of ethane (<2–3 mol%) and hydrogen (<5 mol%) may be present in C–H fluid at <1,200–1,300 K. Despite that, our data strongly suggest that under lithospheric temperatures and pressures (T<1,200 K, P<6 GPa) methane is the major constituent of the C–H fluid. In contrast, the abruptly increased chemical reactivity above 1,200 K provides insight into the behaviour of C-H fluids under deep mantle temperatures and pressures. Observation of the substantial methane dissociation to elemental carbon and molecular hydrogen and/or formation of a mixture of heavier hydrocarbons imply that under the deep mantle pressure–temperature conditions (>6 GPa, >1,500 K) the role of CH 4 in C–H fluid continuously decreases, and at P>24 GPa and T>1,500 K the fluid is likely to be methane-poor, but rich in heavier hydrocarbons. Further experiments are needed to shed light on the respective roles of hydrocarbon phases in fluid under planetary conditions. Our results show a general trend of hydrocarbon reactivity under high pressure and temperature with applications to the Earth’s and icy giant planets’ geochemistry. Generation of oxidized C–O–H fluid (H 2 O–CO 2 ) in the deep Earth is possible through slab devolatilization [29] . Redox interaction of the oxidized C–O–H fluid with reduced ambient mantle [6] can result in the formation of hydrocarbon species in the transition zone or in lower mantle. We argue that reduced C–O–H fluids containing heavy hydrocarbons ascending through the deep mantle (in a plume or convection cell) become carbon-saturated as fluids shift phase composition upon thermodynamic equilibration to lighter hydrocarbons, possessing a higher H/C ratio ( Fig. 5 ). The excess of carbon may be responsible for the formation of ultradeep diamonds, carbides and other carbon-bearing solid phases in the deep Earth. 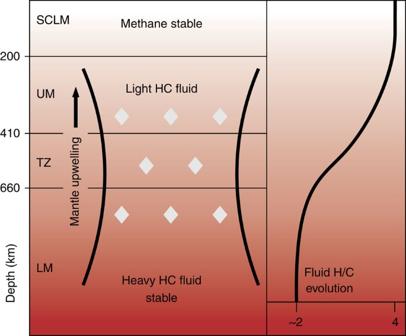Figure 5: A model of C–H fluid evolution in the Earth’s interiors. The composition of the C–H fluid is continuously changing with the depth from lower mantle (LM) via transition zone (TZ) and convecting upper mantle (UM) to subcontinental lithospheric mantle (SCLM). Grey diamonds represent possible loci of diamond precipitation during the ascent of reduced fluid. Figure 5: A model of C–H fluid evolution in the Earth’s interiors. The composition of the C–H fluid is continuously changing with the depth from lower mantle (LM) via transition zone (TZ) and convecting upper mantle (UM) to subcontinental lithospheric mantle (SCLM). Grey diamonds represent possible loci of diamond precipitation during the ascent of reduced fluid. Full size image The observed chemical reactivity of the C–H system and speciation of the reaction products at extreme conditions provides a new insight for the interiors of giant planets such as Uranus and Neptune. These planets are postulated to have mantles consisting of mixture of fluid methane, water and ammonia, where these compounds have a role similar to that of minerals in the Earth’s mantle [1] . The effects of possible formation of mixtures between methane, water and ammonia [30] , [31] and ionization [3] were shown to occur at higher temperatures than those studied in this work. Notwithstanding this, our study offers evidence for chemical reactivity of C–H component of planetary ices, which may also affect positions of planetary isentropes. Therefore, equations of state employed for planetary models should consider chemical reactivity reported in this study. In summary, DAC experiments on CH 4 melting and chemical reactivity in the C–H system show that, at low P–T conditions relevant for the Earth’s crust and uppermost mantle, C–H fluid is represented mainly by methane. In contrast, at T>1,200 K, heavier hydrocarbons, elemental carbon and molecular hydrogen are formed in the C–H system. Thermodynamic equilibration of C–H fluid or hydrocarbons as a part of C–O–H fluid can result in the formation of carbon-bearing solid phases upon a decrease in pressure and temperature in natural environments. This newly documented chemical reactivity of hydrocarbons should also be taken into account in modelling of icy giant planets. Further constrains may be needed to elucidate the role of H 2 O and other potentially important fluid species in the deep Earth or icy giants on methane dissociation, high-pressure equilibria in fluids and ultradeep diamond precipitation. Materials Symmetric DACs equipped with flat (300 μm) and beveled (100 μm) anvils were used to generate pressures up to 80 GPa. Rhenium gaskets (with an initial thickness of 200 μm) were preindented to 40–50 μm, and then the sample cavity was drilled in the centre with a recess to position the couplers apart from the diamond tips. Methane (99.9995%) was loaded into the sample cavity under high pressure (0.2 GPa) using a gas-loading system. A total of 28 methane loadings allowed 41 LH and 13 RH DAC experiments designed either for melting curve measurements, chemical reactivity studies, or both. Resistive heating experiments RH DAC experiments were carried out using a modified high-temperature piston-cylinder Mao-Bell DAC [32] . Two miniature platinum–iridium alloy external resistance heaters were symmetrically mounted around the anvils and their seats, and used to control the temperature up to 1,000 K. A distinct feature of our setup is that the heaters were relatively distant from the pressure-loading mechanism of the DAC, and sapphire discs positioned underneath each anvil seat provided sufficient heat isolation between the hot anvils and the DAC’s body. Our setup enables us to keep the pressure-loading mechanism of the DAC at much lower temperatures than reached in the sample chamber, thus significant pressure stability during RH DAC experiments was achieved. Temperature-corrected ruby barometer [19] was employed to determine pressure in RH experiments; temperature was measured using a S-type thermocouple attached to a diamond anvil near the tip (<±1 K). LH experiments LH experiments were performed by coupling the IR radiation of a fibre laser to Ir and amorphous B absorbers (couplers) positioned in the high-pressure sample cavity and isolated from diamond anvils using the recessed gasket technique [16] ( Supplementary Fig. S3 ). Ir couplers of a different kind were used in experiments designed for melt detection or for chemical reactivity observations. Typically, we used rounded Ir couplers containing three or four holes (being 5–10 μm in diameter). These holes served as sample containers with reduced temperature gradients for in situ Raman spectroscopy during the LH. Pressure was calculated as a mean value between those determined at room temperature before and after LH using a conventional ruby gauge technique [33] . No thermal corrections for pressure were applied. An IR (1,075 nm) Yt-doped fibre laser with improved beam quality [34] was introduced into the optical system using polarizing beam-splitter cubes and focused into a flat top focal spots from two sides of the DAC using the Mitutoyo near-IR × 20 and × 10 long-working distance objective lenses. The focal laser spots were ~ 10–15 μm in diameter, making it possible to heat the coupler around the hole containing the sample. Controlled attenuation of the fibre laser beam was achieved using a combination of the polarizing beam-splitter cube and λ /2 wave plate. Double-sided heating helped to reduce axial temperature gradients. Raman spectroscopy We used custom Raman spectrometers [35] combined with our RH and LH optical systems to collect Raman spectra in the backscattered geometry. The spectra were analyzed with the 460-mm focal length f /5.3 imaging spectrograph equipped with two 1,500 and 300 grooves per mm gratings on the same turret. This feature allows one to combine quick exploratory spectra measurements over a wide spectral range in situ at high temperatures (−4,000–4,000 cm −1 in one spectral window) and accurate measurements with a high spectral resolution (2–4 cm −1 ), which was normally employed on quenched to 300 K samples. In order to reveal a general behaviour of intramolecular hydrocarbon bonds under high pressure, as well as to support identification of newly formed hydrocarbons, we carried out separate pressure runs for ethane, n- hexane and n- docosane up to 40–50 GPa at 300 K. This allowed for the qualitative interpretation of the Raman spectra after quenching. The results of high–pressure Raman studies on short and medium chain alkanes will be published elsewhere. A Witec α-scanning near-field optical microscope was employed for confocal Raman imaging and spot Raman microscopy of synthesized samples studied ex situ outside DAC. A solid-state YAG laser (532 nm) was used to excite Raman scattering. The lateral spatial resolution was as low as 360 nm. Fluid part of the samples was flushed out from DAC upon decompression and only solid reaction products that remained in the sample chamber were examined ( Fig. 3 ). CH 4 characterization and melting in LH experiments Raman microprobe and synchrotron X-ray diffraction were used to verify visual observations and to confirm the liquid state of the vesicles. Methane crystallizes into phase I at 1.7 GPa, into phase A at 5.2 GPa and into phase B at 12–18 GPa [36] . Raman spectra of liquid methane and phase I are very similar and exhibit fundamentals corresponding to symmetric stretching ( ν 1 ), symmetric bending ( ν 2 ) and asymmetric stretching ( ν 3 ) of the C–H bond. The similarity is due to the orientational disorder of CH 4 molecules in the crystal structure of phase I. However, at pressures of >12 GPa, ν 1 and ν 3 fundamentals split as was observed in the Raman spectra [36] , [37] . This splitting is believed to be due to the proton ordering in the crystal lattice [38] . The splitting disappears upon melting, making it possible to use the behaviour of ν 1 and ν 3 modes as a probe for CH 4 melting at pressures of >12 GPa. Synchrotron X-ray diffraction measurements of the vesicle physical state were based both on the appearance of diffuse peak of fluid (structural factor) and disappearance of diffraction spots on two-dimensional (2D) images. Both Raman and synchrotron X-ray data on the physical state of the vesicles additionally confirm them to be fluid. Temperature measurements in LH experiments Characteristic temperatures in LH experiments were measured using the spectroradiometry of the coupler collected from one side of the DAC. The major source of errors in temperature measurements is introduced by approximations for sample emissivity. Namely, the greybody approximation used in this work is known to be a potential source of substantial errors that are on the order of ±100–150 K (refs 39 , 40 ), as sample emissivity is wavelength-dependent and was not characterized as a function of pressure and temperature. Also, there are some minor sources that contributed to the measured melting temperatures. Temperature uncertainties related to the solution of Planck’s equation are relatively small (<1% relative), which is consistent with the results of thorough reports on accuracy of temperature measurements in LH DACs [39] , [40] , [41] . Errors introduced by the optical system were compensated by calibrating the response to tungsten lamp light source. The effects of chromatic aberrations on temperature measurements [42] were minimized by the use of achromatic optics collecting spectroradiometry signals and by a careful selection of a wavelength range for the Planck fitting procedure. Spectral effects induced by the diamond anvil are also minor, as at <2,000 K their contribution to temperature measurement is <1% (ref. 43 ). The total role of minor uncertainties is on the order of ±50 K. In summary, the total uncertainty in temperature measurements can be estimated as ±150–200 K, which is typical for LH DAC studies [20] , [34] , [41] . The temperature measurements are rather accurate above ~ 1,000 K (±150–200 K), whereas below 1,000 K, thermal emission becomes weaker and moves to the IR spectral range, where our radiometry system has a low sensitivity. In some cases, Stokes-to-anti-Stokes intensity ratio was used to compare the temperature of hot methane with the one gained radiometrically. The difference was about 200–300 K and could be due to the contribution of cold methane surrounding the hot spot, which results in lower temperature yields for Stokes-to-anti-Stokes technique. Temperature gradients are large in the LH DAC, but our technique of sequential temperature measurements allows detection of the appearance of small melt vesicles around the heating area, with the melt–solid border only in 2–4 μm away from the hot coupler. The results of finite element calculations of the temperature map in the LH DAC high-pressure cavity show that the coupler is 350 K (±50 K) hotter than the solid–melt border ( Supplementary Fig. S4 ). For simplicity, the cavity has been chosen to have axial symmetry. The coupler has a maximum temperature near 1,150 K at its upper surface. The vesicle of molten material becomes visible if its boundary is at least 2 μm away from the coupler boundary in the radial direction. This corresponds to a melting temperature of ~ 800 K, thus making the temperature difference between that measured radiometrically and of the molten vesicle surface ~ 350 K. We have performed a number of calculations using different values and temperature dependence of the thermal conductivity of methane, which are unknown. Moreover, we took into account the latent heat of melting and the possible large increase of the thermal conductivity of melt. However, this result is quite robust and essentially pressure-independent as this value is mainly determined by experimental geometry and only weakly dependent on the thermochemical parameters of the DAC materials. We used this result to correct the melting temperatures determined in LH DAC experiments: T m = T c −350 K for all pressures. How to cite this article: Lobanov, S. S. et al. Carbon precipitation from heavy hydrocarbon fluid in deep planetary interiors. Nat. Commun. 4:2446 doi: 10.1038/ncomms3446 (2013).